Global migration of influenza A viruses in swine The complex and unresolved evolutionary origins of the 2009 H1N1 influenza pandemic exposed major gaps in our knowledge of the global spatial ecology and evolution of influenza A viruses in swine (swIAVs). Here we undertake an expansive phylogenetic analysis of swIAV sequence data and demonstrate that the global live swine trade strongly predicts the spatial dissemination of swIAVs, with Europe and North America acting as sources of viruses in Asian countries. In contrast, China has the world’s largest swine population but is not a major exporter of live swine, and is not an important source of swIAVs in neighbouring Asian countries or globally. A meta-population simulation model incorporating trade data predicts that the global ecology of swIAVs is more complex than previously thought, and the United States and China’s large swine populations are unlikely to be representative of swIAV diversity in their respective geographic regions, requiring independent surveillance efforts throughout Latin America and Asia. In early 2009, a novel reassortant H1N1 influenza A virus with gene segments from two swine virus (swIAV) lineages emerged in humans, initiating the first influenza pandemic of the 21st century. The virus had a complex genetic composition that had not been previously detected in swine, with six genome segments of North American triple reassortant swine virus origin (PB2, PB1, PA, HA (H1), NP and NS) and two genome segments of Eurasian avian-like swine virus origin (NA (N1) and MP) [1] . Evolutionary analysis of this novel North American/Eurasian reassortant virus indicated that these segments had circulated undetected in swine for at least 8 years (ref. 2 ). The first human outbreak of the pandemic H1N1 virus (pH1N1) occurred in Mexico, and the extent of viral genetic diversity observed in Mexico supports the hypothesis that the virus first emerged there in humans [3] . However, efforts to detect the last common ancestor of the pH1N1 virus in Mexican swine populations have not been successful to date, and the opaque evolutionary history of the pandemic virus in swine highlights the gaps in our understanding of swIAV dynamics at a global scale. In general, influenza viruses in swine are spatially separated into distinct North American and European swIAV lineages, although viruses of North American and European origin both circulate in Asia. Multiple viral lineages co-circulate in North American swine, including (i) ‘classical’ swine viruses, which descend from the 1918 H1N1 pandemic [4] ; (ii) ‘triple reassortant’ swine viruses, which emerged in the mid-1990s with a combination of human, swine and avian segments [5] ; and (iii) ‘delta’ (δ) viruses that are closely related to human seasonal H1 viruses from the early 2000s (refs 6 , 7 ). The main European swIAV lineages include ‘avian-like’ H1N1 viruses that jumped from birds to swine in the 1970s, human-origin H1N1 viruses from the 1980s and human-origin H3N2 viruses that are antigenically described as A/Port Chalmers/1/1973-like [8] . Multiple North American and European-origin swIAV lineages have both been identified in Asian countries [9] , [10] , [11] , [12] . Due to high levels of co-infection, segmental reassortment occurs frequently in swine, such that they are an important reservoir host for influenza virus genetic diversity [9] , [11] , [13] , [14] , [15] , [16] . Live transport is routine in swine farming, and in the United States the transport of millions of swine from Southern to Midwestern regions for end-stage production appears to drive the strongly directional dissemination of swIAVs from Southern US states with high hog production (for example, North Carolina, Texas and Oklahoma) to the traditional centre of swine farming located in the Midwestern ‘corn belt’ [17] . Large numbers of swine also enter the United States from Canada, which has been implicated in the dissemination of other important swine pathogens, including porcine reproductive and respiratory syndrome virus [18] . Intercontinental trade of live swine also occurs, for end-stage production or to acquire female breeding pigs for genetic improvement of swine reproduction or growth traits. Globally, the largest swine population is found in China, where over 450 million hogs reside ( Fig. 1 ). Large swine populations also are found in the United States (>60 million hogs), Brazil (>30 million hogs), Vietnam (>20 million hogs), Germany (>20 million hogs) and Spain (>20 million hogs), among others. 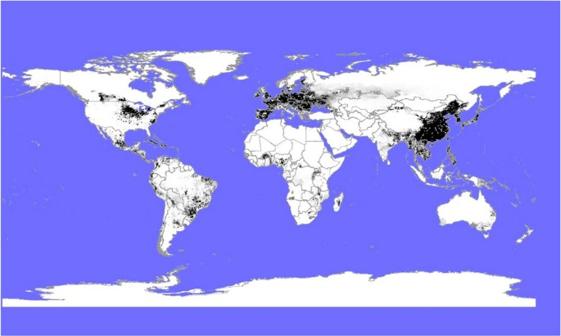Figure 1: Modelled global swine distributions. Digital layers from Gridded Livestock of the World (GLW; version 2.01; ref.50), downloaded from the publically available Livestock Geo-Wiki database (http://www.livestock.geo-wiki.org) and manually edited in QGIS v.1.7.0. Swine densities are represented by the black shading. Figure 1: Modelled global swine distributions. Digital layers from Gridded Livestock of the World (GLW; version 2.01; ref. 50 ), downloaded from the publically available Livestock Geo-Wiki database ( http://www.livestock.geo-wiki.org ) and manually edited in QGIS v.1.7.0. Swine densities are represented by the black shading. Full size image Despite the global nature of both swine farming and swIAV circulation, the patterns and dynamics of the worldwide spread of this economically important virus are unknown. To characterize the phylogeography of swIAVs at a global scale, here we conduct a phylogenetic analysis of 785 whole-genome swIAV sequences collected from 10 countries/regions representing 4 continents, the largest study of its kind undertaken to date. To assess the drivers of viral migration, we compare the phylogeographic patterns with empirical data on live swine trade and swine population sizes. On the basis of these findings, we build a meta-population model to simulate the spatial dissemination of swIAVs at a global scale and to identify the regions that are at a high risk for co-invasion of divergent lineages, increased total genetic diversity and emergence of viruses with pandemic potential. Global migration of swIAVs Phylogenetic analysis revealed that long-distance movement of influenza A viruses between countries and continents has occurred continuously in swine since the 1970s (summarized in Fig. 2 ). Our estimate of 18 international viral migration events is a minimum based on the currently available swIAV sequence data and certainly underestimates the true number. This lower-bound estimate is based on discrete monophyletic groups (defined by country) that are supported by high posterior probabilities (>80), reflecting migration events that led to successful onward transmission. The estimate does not include the much higher number of international viral movements between the United States and Canada or between countries in Europe, which are each considered as meta-populations in our analysis. The estimate also does not consider viral migration events for which only one sequence is available, any viruses that do not form a well-supported clade, or which only partial sequence data were available. 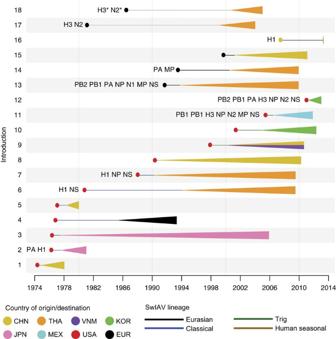Figure 2: Intercontinental migration events of swIAVs. Circles represent the country of origin, based on the estimates summarized in the maximum clade credibility (MCC) tree, and are shaded accordingly. Lines represent the inferred time period of the intercontinental transmission, within a level of uncertainty, inferred from the estimated date of ancestral nodes on the MCC tree. Triangles represent clades resulting from the onward transmission of the introduced viruses, are shaded by the country of destination, and extend as far forward in time as the most recently sampled virus. Numbers of introduction (1–18) correspond to the clade numbers on the phylogenies (Fig. 3andSupplementary Figs 1–7). The asterisks indicate that additional HA and NA swIAV sequence data ware used to estimate the timing of introduction 18. Countries/regions are abbreviated as follows: CHN=China (including Hong Kong SAR and Taiwan), THA=Thailand, VNM=Vietnam, KOR=South Korea, JPN=Japan, MEX=Mexico and EUR=Europe. Figure 2: Intercontinental migration events of swIAVs. Circles represent the country of origin, based on the estimates summarized in the maximum clade credibility (MCC) tree, and are shaded accordingly. Lines represent the inferred time period of the intercontinental transmission, within a level of uncertainty, inferred from the estimated date of ancestral nodes on the MCC tree. Triangles represent clades resulting from the onward transmission of the introduced viruses, are shaded by the country of destination, and extend as far forward in time as the most recently sampled virus. Numbers of introduction (1–18) correspond to the clade numbers on the phylogenies ( Fig. 3 and Supplementary Figs 1–7 ). The asterisks indicate that additional HA and NA swIAV sequence data ware used to estimate the timing of introduction 18. Countries/regions are abbreviated as follows: CHN=China (including Hong Kong SAR and Taiwan), THA=Thailand, VNM=Vietnam, KOR=South Korea, JPN=Japan, MEX=Mexico and EUR=Europe. Full size image Although global surveillance and sequencing of swIAVs has increased markedly in the last 5 years, our timescaled maximum clade credibility (MCC) phylogenies indicate that most intercontinental viral migration events occurred before this increase in surveillance (representative phylogeny of the NA segment is presented in Fig. 3 ; phylogenies for other seven segments are available in Supplementary Figs 1–7 ). Eight of the 18 viral migration events identified in our study were evident on the phylogenies inferred for all eight viral genome segments, indicative of the onward transmission of the full viral genome in the new location (introductions 1, 3, 4, 5, 8, 9, 10 and 15). The consistency of spatial–temporal inferences across these eight segments strengthens inferences of when and where each of these introductions occurred ( Supplementary Table 1 ). Ten viral migration events could only be identified by a subset of genome segments, as at least one segment has been replaced in intervening years by reassortment (introductions 2, 6, 7, 11, 12, 13, 14, 16, 17 and 18). There is no evidence in these data that either of the δ-1 or δ-2 virus lineages that emerged in North American swine in the early 2000s has transmitted to swine on any other continents, despite the high rates of detection in the US swine populations of δ-1 viruses [19] . 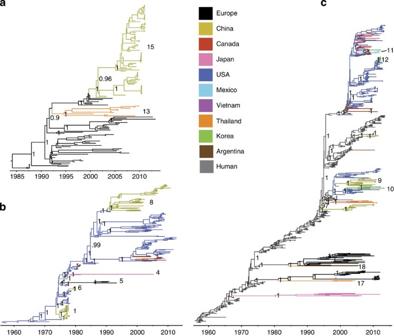Figure 3: Maximum clade credibility (MCC) trees of the NA lineages in swine. Timescaled Bayesian MCC trees inferred for the NA segment for the three major swine virus lineages: (a) avian-origin Eurasian N1 swIAV lineage, the (b) classical N1 swIAV lineage and the (c) multiple human seasonal virus-origin N2 swIAV lineages circulating in swine. Branches of human seasonal H3N2 influenza virus origin are shaded grey inc, while branches associated with viruses from swine are shaded by country of origin: Argentina=brown; Canada=red; China (including Hong Kong SAR and Taiwan)=yellow; Europe=black; Japan=pink; Mexico=light blue; South Korea=green; Thailand=orange; USA=dark blue; Vietnam=purple. Posterior probabilities >0.8 are included for key nodes, and international migration events that are supported by high posterior probabilities and long branch lengths are labelled according toFig. 2. Figure 3: Maximum clade credibility (MCC) trees of the NA lineages in swine. Timescaled Bayesian MCC trees inferred for the NA segment for the three major swine virus lineages: ( a ) avian-origin Eurasian N1 swIAV lineage, the ( b ) classical N1 swIAV lineage and the ( c ) multiple human seasonal virus-origin N2 swIAV lineages circulating in swine. Branches of human seasonal H3N2 influenza virus origin are shaded grey in c , while branches associated with viruses from swine are shaded by country of origin: Argentina=brown; Canada=red; China (including Hong Kong SAR and Taiwan)=yellow; Europe=black; Japan=pink; Mexico=light blue; South Korea=green; Thailand=orange; USA=dark blue; Vietnam=purple. Posterior probabilities >0.8 are included for key nodes, and international migration events that are supported by high posterior probabilities and long branch lengths are labelled according to Fig. 2 . Full size image A consistent global spatial dynamic was observed for swIAVs during 1970–2013, based on both a conservative measure of the strongly supported monophyletic groups ( Figs 2 and 3 and Supplementary Figs. 1-7 ) as well as ‘Markov jump’ counts [20] of the expected number of location state transitions along the branches of the tree. ‘Markov jump’ counts provide a quantitative measure of gene flow between the regions that includes singletons and clusters that may have less phylogenetic resolution ( Fig. 4 , Supplementary Table 2 ). Overall, North America (in this case referring to the United States and Canada) and Europe represent independent viral source populations for the Asian countries sampled in our study: China, Japan, South Korea, Thailand and Vietnam. In contrast, only a single swIAV migration event was observed between North America and Europe (introduction 4). 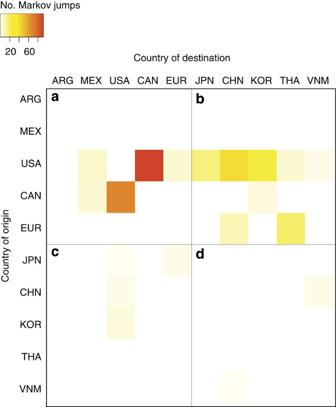Figure 4: Heat-map of swIAV migration between locations. Countries are listed in order of increasing geographical distance from Argentina (ARG). MEX=Mexico, USA=the United States, CAN=Canada, EUR=Europe, JPN=Japan, CHN=China (including Hong Kong SAR and Taiwan), KOR=South Korea, THA=Thailand, VNM=Vietnam. The intensity of the colour (red=high; white=low) reflects the number (no.) of ‘Markov jump’ counts inferred over the totality of phylogenies (all segments, all lineages) from one location to another (asymmetrical). Markov jump counts measure the number of inferred location state transitions, modelled by a continuous-time Markov chain process, that occur along the branches of the phylogeny. For clarity the heat-map has been divided into four sections representing (a) viral migration events within the Americas and between the Americas and Europe; (b) migrations from the Americas/Europe to Asia; (c) migrations from Asia to the Americas/Europe; and (d) migrations between the Asian countries. Figure 4: Heat-map of swIAV migration between locations. Countries are listed in order of increasing geographical distance from Argentina (ARG). MEX=Mexico, USA=the United States, CAN=Canada, EUR=Europe, JPN=Japan, CHN=China (including Hong Kong SAR and Taiwan), KOR=South Korea, THA=Thailand, VNM=Vietnam. The intensity of the colour (red=high; white=low) reflects the number (no.) of ‘Markov jump’ counts inferred over the totality of phylogenies (all segments, all lineages) from one location to another (asymmetrical). Markov jump counts measure the number of inferred location state transitions, modelled by a continuous-time Markov chain process, that occur along the branches of the phylogeny. For clarity the heat-map has been divided into four sections representing ( a ) viral migration events within the Americas and between the Americas and Europe; ( b ) migrations from the Americas/Europe to Asia; ( c ) migrations from Asia to the Americas/Europe; and ( d ) migrations between the Asian countries. Full size image Spatial dynamics of swIAVs in North America . Bidirectional viral migration between Canada and the United States is so frequent (reflected by the extremely high number of Markov jump counts, Fig. 4 ) that Canada and the United States were considered as a single meta-population, similar to Europe ( Fig. 2 ). The higher availability of swIAV sequence data from US swine makes it particularly difficult to distinguish whether an introduction was specifically of the US or Canadian swine origin, and the origin of such introductions is more appropriately characterized as ‘North American’. Using newly generated sequence data from five swIAVs of the H3N2 subtype that were collected in Mexico during 2010–2011 (A/sw/Mexico/SG1442/2010, A/sw/Mexico/SG1444/2011, A/sw/Mexico/SG1447/2011, A/sw/Mexico/SG1448/2011 and A/sw/Mexico/SG1449/2011, accession numbers available in Supplementary Table 3 ), our phylogenetic analysis provides evidence of a single introduction of a H3N2 triple reassortant swIAV from the United States into Mexico that occurred between mid-2005 and mid-2006 (introduction 11, Figs 2 and 3c ). At the time of sampling, all five Mexican swIAVs had acquired at least one pH1N1 segment of the human origin via reassortment, evidence that pH1N1 viruses also have circulated in Mexico’s swine population. Spatial dynamics of swIAVs in Asia Given China’s large swine population and long-term surveillance, it may have been expected that this country (encompassing mainland China, Hong Kong, Taiwan and Macau) would be an important source of swIAV diversity for the neighbouring Asian countries in this study. However, since 1970 there have been 16 swIAV introductions of European or North American origin into Asia, compared with only two swIAV migration events between the Asian countries, and only one definitive introduction of a swIAV from China into another country (introduction 16, Fig. 2 ). Overall, the genetic diversity of swIAVs in Asia derives from five swIAV introductions of European origin and 11 swIAV introductions of North American origin. Six viral introductions from Europe and North America were observed in Thailand, and five introductions were observed in China, including the earliest intercontinental swIAV migration detected to date (introduction 1, Fig. 2 ). In contrast to the frequent exchange of swIAVs across European country borders and across the US–Canadian border, only two swIAV migration events were observed between any two Asian countries. A pair of H1 segments collected in South Korea in 2013 are positioned within a clade of avian-origin Eurasian viruses from China, suggesting China-to-Korea migration (introduction 16, Fig. 2 and Supplementary Fig. 4 ). Closely related North American triple reassortant viruses also were identified in China and Vietnam, suggestive of viral migration between these Asian countries. However, the location state probability for the node representing the common ancestor of the Chinese and Vietnamese clades is too low (ranging from 0.46 to 0.65 across the eight genome segments) to determine whether the North American virus was first introduced to Vietnam and disseminated to China, or vice versa ( Fig. 2 and Supplementary Figs. 1-7 ). Although much of the swIAV diversity in Asia appears to have emerged in the last two decades, the phylogenies suggest long-term circulation of swIAVs in Thailand and Japan, either via imports from North American or European swine in the 1970s and 1980s ( Fig. 2 ) or direct introductions from humans as early as the 1960s ( Fig. 3c ). Long branch lengths and the lack of historical swIAV data from Asian countries make it difficult to infer with confidence the spatial history of older viral lineages in Asia. The relative lack of swIAV surveillance in Thailand before 2000 particularly complicates the estimates of the timing and spatial pathway of the multiple viral introductions from North America and Europe that likely occurred during the 1980s and 1990s (for example, introductions 6, 14, 17 and 18). At this time, there is little evidence of viral dissemination from Japan or Thailand to other Asian countries in our study, despite many decades of potential swIAV circulation. However, the relatively long branches may not reflect a single direct transition between the origin and (final) destination location, and may conceal additional spatial movements during the elapsed time. The evolutionary history of swIAVs in Thailand is also made more complex by the frequency of reassortment involving multiple clades, poorly supported clusters and singletons. Whereas avian-like Eurasian viruses in China are monophyletic and result from a single introduction from Europe (introduction 15), the Thai viruses from this lineage are monophyletic only in the PB2, NP and N1 trees. Our estimate of the two introductions of avian-like Eurasian viruses into Thailand is therefore conservative and likely underestimates the true number (introductions 13 and 14, Figs 2 and 3 , Supplementary Figs 1–7 ). Singletons and unsupported clusters also were observed among South Korean viruses, complicating the estimation of the number of viral migration events into South Korea as well. Importance of live swine trade in the global dispersal of swIAVs We used a generalized linear model (GLM) extension of phylogeographic inference [21] to identify the putative drivers of swIAV migration events inferred from the genetic data. This approach considers single introductions and clusters that may have poor resolution, the uncertainty of which is accommodated by the analysis. The Bayesian model averaging approach found consistent and strong evidence that the amount of asymmetric live swine trade (measured in USD for the years 1996–2012) from one country to another is the dominant driver of the dispersal of SW IAVs globally. This is reflected by the maximal estimated inclusion probability of live swine trade for all six internal gene segments (probability of 1, results for PB2, PB1, PA and NP are presented in Fig. 5 ; results for the shorter MP and NS segments are available in Supplementary Fig. 8 ; the analysis could not be performed on the HA or NA due to the high frequency of human viruses in these phylogenies). Accordingly, viral migration, measured by ‘Markov jump’ counts, was positively correlated with live swine trade volume (USD; ρ =0.52, P =1.5 × 10 −7 , Spearman’s correlation, Supplementary Fig. 9 ). 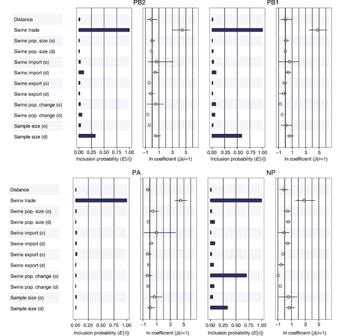Figure 5: The support and contribution of swIAV diffusion predictors among nine countries. Twelve predictors were considered: geographical distance (km), volume of live swine trade, 1996–2012 (USD), swine population size for the years 1969–2010, the total number of imports of live swine during 1969–2010, the total number of swine exports during 1969–2010, the percent change in swine population (pop) size from 1969–2010 and the number of sequences available from a given country for our analysis. ‘O’ refers to the swine population of origin, and ‘d’ refers to the swine population of destination. Support for each predictor is represented by an inclusion probability that is estimated as the posterior expectation for the indicator variable associated with each predictor (E[δ]). The contribution of each predictor is represented by the mean and credible intervals of the GLM coefficients (β) on a log scale conditional on the predictor being included in the model (β|δ=1). SeeSupplementary Fig. 8for MP and NS results. Figure 5: The support and contribution of swIAV diffusion predictors among nine countries. Twelve predictors were considered: geographical distance (km), volume of live swine trade, 1996–2012 (USD), swine population size for the years 1969–2010, the total number of imports of live swine during 1969–2010, the total number of swine exports during 1969–2010, the percent change in swine population (pop) size from 1969–2010 and the number of sequences available from a given country for our analysis. ‘O’ refers to the swine population of origin, and ‘d’ refers to the swine population of destination. Support for each predictor is represented by an inclusion probability that is estimated as the posterior expectation for the indicator variable associated with each predictor (E[ δ ]). The contribution of each predictor is represented by the mean and credible intervals of the GLM coefficients ( β ) on a log scale conditional on the predictor being included in the model ( β | δ =1). See Supplementary Fig. 8 for MP and NS results. Full size image Other potential predictors, including swine population size, contributed little to the observed global spatial patterns, except for the number of sequences of the country of destination (average probability of ~0.5 across the six internal segments). Not only is the effect of live swine trade consistently robust to the inclusion of sample size, the high inclusion probability of live swine trade in cases where the effect of sample size is particularly low (for example, the PA segment) indicates that it is also independent of the sample size. The conditional effect size (the size of the effect conditional on the predictor being included in the model) ranges between ~3 and 5 on a log scale, implying that viral lineage movement probability is several orders of magnitude higher for connections with the highest swine trade compared with connections without trade ( Fig. 5 ). Our GLM analysis could be affected by regional differences in the early establishment of swIAVs, with swIAVs having been potentially seeded later in Asia and decreasing the probability of viral export from Asia. To further explore this hypothesis, we conducted a sensitivity analysis focused on two more recent periods that correspond approximately to the emergence in China of classical North American swIAVs (1990–2013) and avian-origin swIAVs from Europe (2000–2013), using an ‘epoch’ extension of the diffusion model [22] . We find that the volume of live swine is still the only well-supported predictor of viral migration for both the periods ( Supplementary Table 4 ), including when swIAVs are thought to be endemic at high levels in Asia as well as Europe and North America. The relatively low number of highly supported migration events during 2000–2013 ( Fig. 2 ), transitions involving singleton viruses or clades that do not have high bootstrap support also contribute to the signal over this restricted time period, including migrations across the relatively porous US–Canada border and between the US/Canada and South Korea. Predicted spatial dissemination of swIAVs To explore how the global network of live swine trade may drive movements of swIAVs beyond the 10 countries for which whole-genome sequence data were available, we used data on pairwise live swine trade between the 146 countries to simulate the patterns of viral dissemination under different epidemiological scenarios. 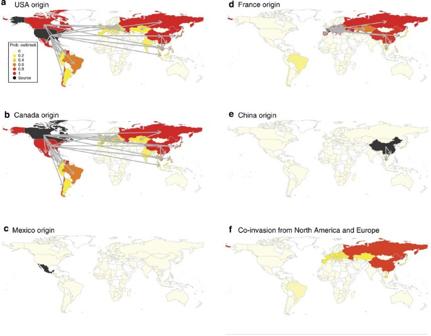Figure 6: Maps of the simulated spread of influenza viruses via live swine trade flows. Simulated spread of an influenza virus from five seed countries (shaded in black) to 146 countries for which live swine trade is available from the United Nations Commodity Trade Statistics Database (available athttp://comtrade.un.org) (a–e). The probability (prob.) of an outbreak in the invaded country is shaded from white (probability of 0) to red (probability of 1). The probability of co-invasion by both a virus seeded in North America (Canada and the United States) and Europe also is shaded from white (probability of 0) to red (probability of 1;f). Arrows represent the direction of viral dissemination for countries with a probability of an outbreak >0.25 (seeSupplementary Table 5for a complete list of all outbreak probabilities by country). Figure 6 explores the predicted spatiotemporal spread of a new swIAV lineage that hypothetically originates in swine in one of five countries with large swine populations: Canada, China, France, Mexico and the United States. These predictions are largely consistent with the spatial movements observed in the genetic data, with a high probability of viral export from the United States and Canada into Asia, and from Europe to Asia, whereas epidemics originating from China have low probabilities of onward dissemination to other countries ( Supplementary Table 5 ). In addition, we identified predicted connections with countries not sampled in our study, including swIAV migration from the United States and Canada to many countries in Latin America, as well as Russia, Kazakhstan, Malaysia and Singapore. Interestingly, our model suggests that a virus seeded in Mexican swine is comparatively less likely to disseminate to swine in other countries, including the United States. Figure 6: Maps of the simulated spread of influenza viruses via live swine trade flows. Simulated spread of an influenza virus from five seed countries (shaded in black) to 146 countries for which live swine trade is available from the United Nations Commodity Trade Statistics Database (available at http://comtrade.un.org ) ( a – e ). The probability (prob.) of an outbreak in the invaded country is shaded from white (probability of 0) to red (probability of 1). The probability of co-invasion by both a virus seeded in North America (Canada and the United States) and Europe also is shaded from white (probability of 0) to red (probability of 1; f ). Arrows represent the direction of viral dissemination for countries with a probability of an outbreak >0.25 (see Supplementary Table 5 for a complete list of all outbreak probabilities by country). Full size image We also used our model to estimate the probability of co-invasion of European and North American swIAVs lineages, illustrating the potential for reassortment between the lineages of European and North American descents, of the kind that generated the 2009 pH1N1 virus. Overall, co-invasion is strongly regionalized, with the highest probability in East and South-East Asian countries, particularly China, South Korea and Russia ( Fig. 6 , Supplementary Table 5 ). Conversely, South Asia, the Middle East, Africa and Australia exhibited a low probability of invasion by each of these lineages. Mid-level probabilities were found in regions with a high probability of invasion by only one of the two lineages (that is, the North American lineage in the Americas and the Eurasian lineage in Europe). Interestingly, these simulations reveal a low probability of co-invasion in Mexico, where pH1N1 first emerged in humans, owing to the low probability of invasion by a European swine virus in Latin America. The unknown origins of the swine virus that begot the 2009 H1N1 pandemic underscores the importance of understanding how influenza A viruses evolve in swine at a global scale, including regions where swIAV surveillance is lacking. Our expansive phylogenetic analysis of global swIAV sequence data demonstrates the importance of the asymmetrical nature of the global live swine trade on the global ecology and evolution of swIAVs. Using a phylogeographic GLM approach to assess the strength of specific predictors, we determine that the size of a country’s swine population is not a major factor in the rate of viral export to other countries. As a notable case in point, China, which hosts the world’s largest swine population, does not appear to be a major source of the viral diversity observed in other Asian countries ( Fig. 4d ). Rather, Japan, Thailand, Vietnam and South Korea independently imported novel viruses from Europe and North America ( Fig. 4b ), most likely via long-distance live swine trade. The reported pattern of swIAV dissemination is a reverse of a model proposed for the global spread of A/H3N2 seasonal influenza viruses in humans, in which a highly connected network of South-East Asian countries, including China, acts as a key source of viruses for Europe, North America and other continents [21] , [23] , reflecting differences in the disease and mobility patterns of humans and swine. These findings have important implications for swIAV surveillance strategies, as the relatively low levels of viral gene flow between Asian countries means that no single country in Asia can serve as a proxy for the region, including China’s large swine herds. The extent of viral genetic diversity in Thailand highlights the importance of enhancing surveillance throughout South-East Asia, including countries not sampled in our study, such as Malaysia, Indonesia, Singapore, Laos and Cambodia, and undersampled countries such as Thailand, Vietnam, Japan and South Korea. Furthermore, Russia emerged as a hotspot for invasion and co-invasion of divergent lineages in our simulations, and yet Russia has no publicly available whole-genome swIAV sequences. The limited number of sequences from Asian countries other than China (particularly via Hong Kong, the final destination of large numbers of hogs from mainland China) reduces our ability to detect viral migration events within Asia, particularly those that do not transmit onward in swine for many years. However, the high number of viruses identified in Asia that were of North American and European origin indicates that sample bias alone cannot explain the lack of viral exchange observed between the Asian countries. Analysis of larger, less-constrained data sets including all available HA swIAV sequences from Asia identified several additional viral migration events from Europe and North American swine into Asia, but only limited evidence for one additional putative connection between two Asian countries ( Supplementary Figs. 10-11 ). However, all inferences of spatial connections must be interpreted within the context of the many countries that are unsampled and undersampled, and long branches may conceal additional spatial movements between the origin and (final) destination location. It is important to note that our study focused only on the international dissemination of swIAVs, and did not consider the probability of initial emergence of an epidemic within a country, which is likely to be influenced by numerous local factors related to national swine farming practices, including the size and density of farms, movements of pigs within countries and the opportunities for interspecies transmission. As demonstrated previously, the dynamics of outbreaks within a large country like the United States can be complex, with different regions acting as source and sink populations for viral diversity [17] . Novel IAVs of human origin have emerged repeatedly in swine in countries in North America, South America, Asia and Europe, suggesting that swine populations in these regions can sustain new epidemics [24] . The extent of viral export from a country of origin is a product of both the national prevalence of circulating swIAVs and the volume of live swine export. In this study, we were unable to assess whether geographic differences in the prevalence of swIAVs affect large-scale viral migration, as population-level virological and serological data indicative of swIAV prevalence are available only from a limited number of study sites and time periods that are unlikely to be sufficiently representative for a global study. We therefore recognize that there are scenarios where live swine trade alone would not be a good predictor of viral migration. For example, if the major exporters of live swine (North America and Europe) did not have large endemic swIAV populations, then live swine trade alone would not be a good predictor of viral migration. This does not appear to be the case, as North America and Europe have long histories of endemic swIAV circulation and the highest volumes of outgoing international live swine trade. The apparent association between viral endemicity and trade export may not be a coincidence, as the features that enable countries in Europe and North America to export high volumes of live swine (that is, large-scale commercial swine production) also are likely to be conducive to sustained endemic swIAV transmission. Finally, our analysis did not consider swine influenza vaccine use, which is highly heterogeneous within and between countries, and would be an important, albeit challenging, factor to integrate into future studies that consider the interaction between the national prevalence of swIAVs, the structure of swine industries, and the global spatial dynamics of trade and viral migration. Although it is not possible at this time to incorporate empirical data on historical differences in swIAV prevalence by region, we were able to explore the interaction of influenza virus prevalence and trade volume using our simulation model. Of particular interest was the question of whether the low levels of viral export from Asia observed in our study could be an artifact of the historically lower levels of endemic swIAV activity in Asia. As a consequence, viral exports from Asian countries might be expected to rise in the future as swIAVs become endemic at higher levels throughout the region. There was no support for this hypothesis, as our simulations predicted very low rates of viral export from China to other countries even when the prevalence of swIAVs in China is set unrealistically high (for example, 58% of the Chinese swine were infected when R 0 =1.5). Our simulations predicted low rates of swIAV export from Japan and Thailand under similar transmissibility scenarios ( Supplementary Fig. 12 ), with the exception of viral dissemination from Thailand to Cambodia, as these countries are trade partners. These predictions are consistent with our observation from the genetic data that swIAVs could have circulated in Japan and Thailand for many decades without substantial onward dissemination to other Asian locations sampled in our study. In addition, a sensitivity analysis of the GLM model, limited to the more recent 1990–2013 and 2000–2013 periods where swIAVs were established in Asia, lends further support for the importance of trade ( Supplementary Table 4 ). Overall, our findings suggest that viral exchange between Asian countries with low levels of trade is unlikely to increase in the future, regardless of the potential increases in endemic swIAV activity in the region as farming practices are modernized and swine farms become larger. Despite the importance of swine trade in the global ecology of swIAVs, it should be noted that humans may be equally, if not more, important in disseminating IAV diversity to swine herds globally [25] . Even in the absence of international swine trade, swIAVs of human origin would likely still circulate in the majority of countries in our study, including in Asia. Quarantine and other restrictions in international trade may have the potential to reduce the genetic diversity of swIAVs, but are not likely to prevent swIAVs from circulating in a country’s swine population (Australia is a case in point [26] ). The frequency of human-to-swine transmission has been even more apparent since the 2009 H1N1 pandemic, and humans have disseminated pH1N1 viruses to swine in numerous countries that had not previously reported IAV activity in swine, including Australia [26] , [27] , Brazil [28] , [29] , India [30] , Cameroon [31] , Mexico [32] , Nigeria [33] , Sri Lanka [34] and several countries in Europe [35] , [36] , [37] . Unfortunately, these new data did not advance our understanding of the evolution of the pH1N1 virus during the many years of undetected circulation in swine before 2009. Given that the human pandemic likely emerged in Mexico [3] , the most parsimonious explanation is that the pH1N1 virus transmitted from swine to humans in Mexico or a nearby locality. However, extremely little swIAV sequence data are available from swine in Mexico and other parts of Latin America, and Eurasian viruses have not been detected in any part of the Americas to date. Our simulation model provides a quantitative indicator of where the reassortment event that produced the pH1N1 virus in swine was most likely to have occurred, based on the probability of invasion with both North American and European viruses. Given limitations in our model, including the lack of information on within-country dynamics and the likelihood of initial viral emergence within seed countries, we consider the relative ranking of probabilities to be more important than their absolute values. To date, Asia is the only region where any reassortant viruses containing both North American and Eurasian virus segments have been detected [38] , consistent with our simulations, which show a high probability of co-invasion by both North American and Eurasian swine lineages in China, South-East Asia and Russia. However, it remains unclear how a reassortant virus that most likely emerged in swine in Asia caused its first outbreak in humans in Mexico. Given the lack of south-to-north swine trade flows in the Americas, some swIAV lineages are likely to be exclusive to Latin America [39] , [40] and not reach the United States or Canada. Strengthened surveillance in Latin America is needed to gain a better understanding of swIAV diversity in the region. Finally, we have focused our study on the global dynamics of influenza A viruses in swine, but our findings invite investigation of how trade, quarantine and swine farming practices affect the spatial dynamics of other globally dispersed swine pathogens, such as porcine reproductive and respiratory syndrome virus and the porcine epidemic diarrhoea virus that emerged in the United states swine herds in 2013. Modelling studies rooted in pathogen sequence information, demographics and mobility data have the power to inform global surveillance and control strategies for major animal and human disease threats. Influenza virus sample preparation Influenza A virus samples collected from swine via routine diagnostic submissions for the years 2002–2011 were randomly selected from the existing influenza virus archive at the University of Minnesota Veterinary Diagnostic Laboratory (UMVDL). These samples were chosen to best represent this time period and the three main geographical regions of the US hog production: the Southeast region (US states of Alabama, Georgia, Kentucky, North Carolina, Tennessee and Virginia), South-central/west region (Arkansas, Colorado, New Mexico, Oklahoma and Texas) and Midwest region (Iowa, Illinois, Indiana, Kansas, Minnesota, Missouri and Nebraska). Samples from swine in Canada (2005–2011) and Mexico (2010–2011) also were selected from UMVDL, as available. Original specimen material (nasal swab supernatant or lung tissue homogenate stored at −80 °C) were aliquotted from the archived samples and sent to the J. Craig Venter Institute (JCVI) in Rockville, MD for sequencing. Influenza virus genome sequencing The complete genomes of 240 influenza viruses collected from North American swine were sequenced at JCVI. Viral RNA was isolated using the ZR 96 Viral RNA kit (Zymo Research Corporation, Irvine, CA, USA). The influenza A genomic RNA segments were simultaneously amplified from 3 μl of purified RNA using a multi-segment reverse transcription-PCR strategy (M-RTPCR) [41] . The M-RTPCR amplicons were sequenced using Nextera Library construction using the MiSeq platform (Illumina Inc., San Diego, CA, USA). In addition, M-RTPCR amplicons were sheared for 7 min and Ion Torrent compatible barcoded adapters were ligated to create 200 base pair libraries that were purified and sequenced using Ion Torrent (Life Technologies, Grand Island, NY, USA). All data sequenced for this study were submitted to the Influenza Virus Resource at the National Center for Biotechnology Information’s GenBank [42] , and accession codes are available in Supplementary Table 3 . Phylogenetic analysis In addition to the sequences generated for this study, whole-genome sequences from influenza A viruses collected in swine globally during 1960–2013 were downloaded from the Influenza Virus Resource at GenBank [42] . Viruses were removed that (a) had truncated sequences, (b) were of avian origin with no evidence of circulation in swine, (c) had unknown geographic origin or (e) had evidence of lab errors (assessed by root-to-tip divergence using the program Path-O-Gen v1.3). Due to the disproportionately large number of swIAV sequences from the United States for the years 2009–2013, 100 of these were randomly subsampled. Sequence alignments were constructed for each of the six internal gene segments (PB2, PB1, PA, NP, MP and NS) and for the H1, H3, N1 and N2 antigenic segments separately using MUSCLE v3.8.31 (ref. 43 ), with manual correction in Se-Al v2.0 (available at http://tree.bio.ed.ac.uk/software/seal/ ). Phylogenetic trees were inferred using the neighbor-joining method available in PAUP v4.0b10 for each of the 10 alignments (available at http://paup.csit.fsu.edu/ ). For the PB2, PB1 and PA segments, each virus was categorized as belonging to one of the following lineages: (a) classical swine virus lineage, (b) triple reassortant (‘trig’) lineage, (c) avian-origin Eurasian swine lineage, (d) the pH1N1 lineage that emerged in humans in 2009 and transmitted from humans to swine globally during 2009–2013 or (e) related to human seasonal influenza A viruses. For the NP, MP and NS segments, each virus was categorized as (a) classical, (b) avian-origin Eurasian, (c) pandemic or (d) human seasonal. No ‘trig’ category exists for the NP, MP and NS segments because triple reassortant viruses contain classical virus NP, MP and NS segments acquired through reassortment. For the H1 and N1 segments, each virus was categorized as (a) classical, (b) avian-origin Eurasian, (c) pandemic or (d) human seasonal virus origin. All H3 and N2 segments belonged to the same category: human seasonal H3N2 virus related. The sequence alignment for each segment was further divided into each of these lineages. For the PB2, PB1, PA, NP, MP, NS and N1 segments, very few (<10) viruses were found to be of recent human seasonal virus origin, which is consistent with previous findings [24] , so these data sets were excluded from further analyses. The pH1N1 viruses that have been recently transmitted from humans to swine since 2009 remain spatially structured by country (or continent), with little evidence of long-distance migration between the continents [44] , and therefore sequences of pH1N1 origin were not included in further analyses. Similarly, no global migration was observed among N1 swIAV sequences that were closely related to human seasonal H1N1 viruses, and they were excluded from the study. In total, 22 segment- and lineage-specific data sets were included in the analysis ( Supplementary Table 6 ; Supplementary Data 1 ). For the H3, N2 and H1 human-like (δ) lineages, human seasonal influenza virus H3, N2 and H1 sequences also were included as background. To reduce the impact of sample bias, additional phylogenies were inferred using all available full-length swIAV H1 and H3 sequence data from Asia, which included an additional 206 swIAVs from China, South Korea, Thailand and Japan for the classical H1 segment, 191 swIAVs from China for the avian-origin Eurasian H1 segment and 230 swIAVs from China, Thailand, Japan, Mongolia, South Korea and Indonesia for the human seasonal virus origin H3 segment. Phylogenetic relationships were inferred for each of the 22 data sets separately using the timescaled Bayesian approach using MCMC available via the BEAST v1.8.00 package [45] and the high-performance computational capabilities of the Biowulf Linux cluster at the National Institutes of Health, Bethesda, MD ( http://biowulf.nih.gov ). A relaxed uncorrelated lognormal molecular clock was used, with a flexible Bayesian skyline plot demographic model (10 piece-wise constant groups) and a general-time reversible model of nucleotide substitution with gamma-distributed rate variation among sites. For viruses for which only the year of viral collection was available, the lack of tip date precision was accommodated by sampling uniformly across a 01-year window from January 1st to December 31st. The MCMC chain was run separately three times for each of the data sets for at least 100 million iterations with subsampling every 10,000 iterations, using the BEAGLE library to improve computational performance (ref. 46 ). All parameters reached convergence, as assessed visually using Tracer v.1.6, with statistical uncertainty reflected in values of the 95% highest posterior density. At least 10% of the chain was removed as burn-in, and runs for the same lineage and segment were combined using LogCombiner v1.8.00 and downsampled to generate a final posterior distribution of 1,000 trees that was used in subsequent analyses. The phylogeographic analysis considered 10 locations: Argentina, Canada, China, Europe, Japan, Mexico, Thailand, the United States, South Korea and Vietnam. All viruses from Europe (our study included swIAV data from Belgium, Czech Republic, Denmark, France, Germany, Italy, Netherlands, Poland, Spain and the United Kingdom) were categorized into a single spatial category due to the high level of influenza virus mixing within Europe ( Supplementary Fig. 13 ) and the relatively low level of sampling of individual countries. Similarly, we considered Hong Kong viruses to be part of China based on genetic similarities. The location state was specified for each viral sequence, allowing the expected number of location state transitions in the ancestral history conditional on the data observed at the tree tips to be estimated using ‘Markov jump’ counts [20] , which provided a quantitative measure of asymmetry in gene flow between regions (a representative XML file used in the analysis is provided in Supplementary Data 2 ). For computational efficiency the phylogeographic analysis was run using an empirical distribution of 1,000 trees (ref. 21 ), allowing the MCMC chain to be run for 25 million iterations, sampling every 1,000. A Bayesian stochastic search variable selection was employed to improve the statistical efficiency for all data sets containing >4 location states. Maximum clade credibility trees were summarized using TreeAnnotator v1.8.0 and the trees were visualized in FigTree v1.4.2. Testing predictors of global swIAV migration A GLM [21] parameterization of the discrete phylogeographic diffusion model was employed to estimate the contribution of potential predictors to the migration patterns of swIAVs (a representative XML file used in the analysis is provided in Supplementary Data 3 ; the R code used to summarize the estimates is provided in Supplementary Data 4 ). First, the trade value (USD) for live swine trade between countries (asymmetric) for the years 1996–2012 was obtained from the United Nations’ Commodity Trade Statistics Database (available at http://comtrade.un.org , accessed March 20, 2014) ( Supplementary Data 5 ). For the purposes of our study, we calculated the total trade value for each country. Data from all European countries were aggregated within the category ‘Europe’, and the data from mainland China, Macao SAR and Hong Kong SAR were aggregated within the category ‘China’. Second, estimates of the number of live swine by country and the total number of live swine imports and exports per country were obtained for a longer time period (1969–2010) from the Food and Agriculture Organization (FAO) of the United Nations Datasets repository (available at http://data.fao.org/datasets , accessed March 21, 2014) ( Supplementary Table 7 ). Again, data were aggregated across years and for Europe as well as for China. Although there is variance in trade volumes between the years, some of which may also reflect variance in reporting, consistent differences in trade volume were evident among countries across years ( Supplementary Fig. 14 ). Further, we estimated the country-specific percentage change in the pig population over the study period (ratio of the numbers of live swine in 1969 versus 2010) as an additional putative predictor of swIAVs migration. All the predictors were log-transformed and standardized before their specification in the GLM parameterization. We performed the GLM analysis separately for each of the six internal gene segments (PB2, PB1, PA, NP, MP and NS) and jointly for all three swIAV lineages (avian-origin Eurasian, triple reassortant and classical) for each segment. We achieve this, for each segment, by sharing a single GLM-diffusion model across the independent evolutionary histories of the three viral lineages. For the NP, MP and NS segments only two lineages were included, as the triple reassortant lineage is an extension of the classical lineage for these three segments. We also excluded Argentina from the GLM analysis because no viral migration was observed between Argentina and any other country in our study. In addition, to explore the effect of regional differences in the early establishment of swIAVs we used an ‘epoch’ extension of the diffusion model [22] for two periods that correspond approximately to the emergence in China of classical North American swIAVs (1990–2013) and avian-origin swIAVs from Europe (2000–2013; representative XML file is provided in Supplementary Data 6 ). Meta-population model simulating the global spread of swine influenza Next, we built a meta-population model to simulate the global spread of swIAVs and identify the potential geographical hotspots for reassortment between viruses originating from different regions, which may generate novel viruses with pandemic potentials. We employed a stochastic patch-based SIR model adapted from an earlier model for the global diffusion of human influenza [47] . Each patch represents the swine population of an individual country, and patches are linked based on the live swine trade movements. To calibrate the model, we obtained swine population sizes and pairwise between-country trade information for 146 countries reporting to FAO during 1969–2010 ( http://data.fao.org/datasets ; Supplementary Table 7 , Supplementary Data 5 ), which coincides with the study period considered for phylogenetic analysis of swIAVs. We used the averages of swine population sizes and pairwise trade volumes throughout the study period for model simulations. The influenza simulation model is as follows. Let S , I and R denote vectors representing the number of susceptible, infected and recovered swine at any time point in each of the 146 countries studied. We let μ =1/5 denote the daily probability that an individual recovers (so that the infectious period is 5 days [48] , [49] ), and β I the daily per capita rate of infection from infectious individuals within the same country. Here β varies between countries; it is a vector scaled such that the effective reproduction number= β N / μ is the same in all countries, where N is the vector of swine population sizes. We use an R 0 of 1.5 in main analyses, consistent with limited information on swine influenza dynamics. [48] , [49] The per capita rate of contacts with infectious swine from other countries is given by G * I , where G is a 146*146 coupling matrix representing between-countries swine fluxes. To build G , we first create T , a 146*146 matrix with off-diagonal elements based on empirical live swine trade and zeros along the diagonal. We then rescale T by the estimated trade coefficients of the phylogeographic GLM model, as the GLM model suggests that the relationship between trade and viral migration is not linear (but results are qualitatively similar with no rescaling). Following the past work [47] , the rescaled matrix T ′ is then tuned by a free parameter, c , which governs the amount of international versus domestic contacts between swine, while at the same time allowing the conversion of empirical swine trade data (provided in $ amount by FAO) into actual population movements. Tuning parameter c allows obtaining realistic time course of infection, with global epidemics lasting between several months to several years, in line with (limited data available on) the global spread of past swine outbreaks. Our final coupling matrix is G = c T ′, where c is such that the maximum element of the coupling matrix is <10 −3 . We use a spatially extended chain-binomial system to update the progression of the epidemic in each patch [47] : Here, W t is the daily incidence of swine influenza (that is the number of new cases), and V t is the number of new ‘recovereds’. In simulations, the epidemic is initialized by infecting five swines in a predetermined seed country; we explored various scenarios with seeds in countries of the Americas, Europe and Asia. After the first infection occurs in each country, we draw from a multinomial distribution using a normalized vector G*I to determine the source of infection. For each scenario, involving a given source country (for example, US, Canada, UK, France and China), we run 1,000 simulations, allowed to run over a 3-year time period and assess the probability of swine flu invasion in each non-source country, and its most likely source of infection. We conducted sensitivity analyses with higher and lower values of the free parameter c and R 0 , which mostly affected the time course of the global epidemic and the synchronicity of epidemics across locations, but did not change markedly the identification of hotspots countries for the onward spread. To explore the probability of reassortment between viruses originating from North America and Europe, we ran 1,000 independent simulations of epidemics starting in North America (USA and Canada), and in each the 10 European countries with largest swine populations, and compute the co-invasion probability in country i , following: P.coinv .i =[1−Π j source countries in North America (1− p.inv i,j )] * [1−Π k source countries in Europe (1− p.inv i,k )], where p.inv i,k is the probability that country i is invaded when the outbreak is seeded in country k . Estimates were then used to produce risk maps for swIAV invasion and co-invasion using the rWorldmap package available in the R software ( http://www.r-project.org/ ). Accession codes : All sequences from swine influenza A viruses that were generated and used in this study have been deposited in the GenBank database with the accession codes AHB20822 to AHB20891 , AHB20919 to AHB23256 , AHB23664 to AHB23860 , AHB24418 to AHB24833 and AHB82076 to AHB82086 . How to cite this article: Nelson, M. I. et al . Global migration of influenza A viruses in swine. Nat. Commun. 6:6696 doi: 10.1038/ncomms7696 (2015).